Perceiving invisible light through a somatosensory cortical prosthesis Sensory neuroprostheses show great potential for alleviating major sensory deficits. It is not known, however, whether such devices can augment the subject’s normal perceptual range. Here we show that adult rats can learn to perceive otherwise invisible infrared light through a neuroprosthesis that couples the output of a head-mounted infrared sensor to their somatosensory cortex (S1) via intracortical microstimulation. Rats readily learn to use this new information source, and generate active exploratory strategies to discriminate among infrared signals in their environment. S1 neurons in these infrared-perceiving rats respond to both whisker deflection and intracortical microstimulation, suggesting that the infrared representation does not displace the original tactile representation. Hence, sensory cortical prostheses, in addition to restoring normal neurological functions, may serve to expand natural perceptual capabilities in mammals. Most sensory neuroprosthetic systems aim to restore function within the same modality as a pre-existing sensory deficit. For instance, cochlear implants restore auditory function [1] , and stimulation along the visual pathway can restore visual function [2] , [3] . In some cases, however, it might be necessary to augment, rather than simply restore, the usual function of a sensory area [4] , [5] . For instance, in people that suffer permanent damage to the visual cortex, we might ask the somatosensory cortex to take over some of the roles of the visual system. Such cross-modal plasticity has been demonstrated in juvenile animals [6] , [7] , [8] . For example, rewiring experiments in newborn ferrets have shown that when visual inputs are rerouted to the auditory cortex, the auditory cortex acquires many anatomical and functional properties of the visual cortex [7] , [8] , and even mediates visually guided behaviour [8] . Such results suggest that the function of a primary sensory area can dramatically change depending on the type of input it receives from the environment [9] , [10] . To date, however, the literature lacks a clear demonstration of such functional plasticity in normal adult mammals. This would require that the adult brain be plastic enough to extract novel information embedded within pre-existing representations, and use this information to generate appropriate behaviours. In the present study, we test whether adult rats can incorporate a novel sensory modality into their perceptual repertoire. Specifically, we examined whether adult rats could learn to discriminate among infrared (IR) sources after we coupled the output of a head-mounted IR detector to electrical microstimulators in the whisker representation of S1. We discovered that, after training with this sensory prosthetic device, adult rats learned to navigate their IR world as if they had acquired a novel distal sensory modality. Behavioural performance We initially trained six rats on a simple visual discrimination task. Rats were placed in a circular chamber that included three reward ports ( Figs 1a ). On each trial, a visible LED was activated in one of the ports, and rats were rewarded with water for poking their nose in that port. Once they reached criterion on this task (70% correct, after 25±5 days (mean±s.e.m. )), we surgically affixed an IR detector to the rat’s head, and implanted stimulating microelectrodes in the whisker region of S1 cortex ( Figs 1c ). 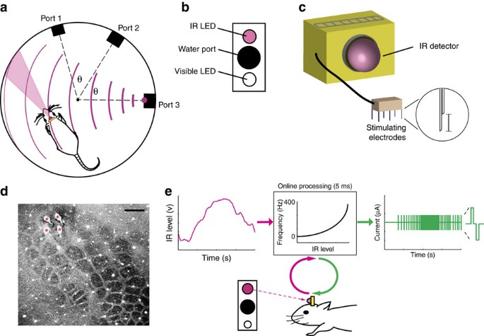Figure 1: Methods. (a) Set-up of the IR behaviour chamber. Three reward ports line the walls of the circular chamber. The proximity of the ports to one another is indicated by the angleθ.The rat has an IR detector (red) affixed to its head, and the cone emanating from the detector represents the area within which it will respond to IR stimuli. The red lines emanating from port 3 represent the IR signal emitted from that IR source. (b) Arrangement of each reward port, which includes a recess with a water spout, an IR LED above, and a broad-spectrum visible LED below. (c) Design of stimulating electrodes (see Methods for details). The inset shows how each stimulating electrode pair is configured in the array (scale bar, 300 μm). (d) Example of electrode placement. Cytochrome oxidase-stained barrel field shows the location of four stimulating electrodes. Each penetration is indicated with a red asterisk. Reference line: 500 μm. (e) Coupling IR levels with ICMS. On each trial, the IR light turns on, which activates the IR detector that is mounted on the rat’s head. Processing converts the detected IR level into a stimulation frequency. This value is sent to the microstimulator, which produces the desired current pulses. The inset on the right-hand-side illustrates the structure of each biphasic waveform in the pulse train. Figure 1: Methods. ( a ) Set-up of the IR behaviour chamber. Three reward ports line the walls of the circular chamber. The proximity of the ports to one another is indicated by the angle θ. The rat has an IR detector (red) affixed to its head, and the cone emanating from the detector represents the area within which it will respond to IR stimuli. The red lines emanating from port 3 represent the IR signal emitted from that IR source. ( b ) Arrangement of each reward port, which includes a recess with a water spout, an IR LED above, and a broad-spectrum visible LED below. ( c ) Design of stimulating electrodes (see Methods for details). The inset shows how each stimulating electrode pair is configured in the array (scale bar, 300 μm). ( d ) Example of electrode placement. Cytochrome oxidase-stained barrel field shows the location of four stimulating electrodes. Each penetration is indicated with a red asterisk. Reference line: 500 μm. ( e ) Coupling IR levels with ICMS. On each trial, the IR light turns on, which activates the IR detector that is mounted on the rat’s head. Processing converts the detected IR level into a stimulation frequency. This value is sent to the microstimulator, which produces the desired current pulses. The inset on the right-hand-side illustrates the structure of each biphasic waveform in the pulse train. Full size image After this surgical procedure, we returned the animals to the same chamber, where they had to learn to perform the same task using IR light, which is invisible to rats (see Methods for details on the task and training) [11] . To allow the rats to perceive IR light levels, the value of the IR detector output was converted into a pattern of electrical stimulation in S1, with stimulation frequency updated every 50 ms depending on the IR intensity detected ( Fig. 1d ). Electrical stimulation frequency increased as rats approached, or oriented their heads toward, an IR source (see Supplementary Movie 1 ). Note that such electrical stimulation in S1 is known to induce some type of tactile sensation in humans [12] and monkeys [13] . It took 26±6 days for all six implanted rats to learn to discriminate among the IR sources at or above the criterion used in the initial visual task (>70% correct). While training with their new IR gear, rats underwent clear changes in behavioural strategy. At first, they did not associate intracortical microstimulation (ICMS) with the task, and would poke randomly in the reward ports, occasionally scratching their faces in response to microstimulation. Eventually they learned to actively forage through the behaviour chamber, sweeping the IR sensor on their heads back and forth to sample their IR world (see Supplementary Movies 2 , 3 , 4 ). Quantitatively, the rats’ performance increased from 41±6 to 93±2% correct during learning ( Fig. 2a ), and their best single-session performance averaged 95±3% correct. Their behavioural latency on correct trials (the time between stimulation onset and poking in the correct reward port) decreased significantly as they improved at the task (latency dropped from 2.3±0.01 to 1.3±0.03 s; Fig. 2b ; r =−0.71; P =1.9017 × 10 −11 ( t -test)). 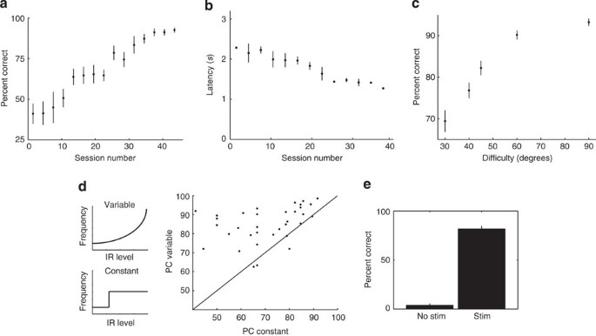Figure 2: Rats discriminate among IR sources using graded stimulation frequencies. (a) Learning curve for IR-only trials. Graph shows percentage of correct trials as a function of session number (130 sessions in four rats). Black circles/lines indicate mean/s.e.m. for blocks of three sessions. (b) Latency decreases as rats learn the task. Scatter plot of latency on IR-only trials, using same conventions as panela(data are from 66 sessions in two rats). (c) Discrimination performance varies with angle between ports. Plot shows percentage of correct trials versus task difficulty (angle between ports). Data are from 100 sessions in two rats. (d) Performance degrades when stimulation frequency is constant rather than variable. Plot on the right shows performance on trials in which the stimulation frequency is variable (top left inset) versus held constant (bottom left inset). Data are from 34 sessions in two rats. (e) When stimulation is turned off, performance is abolished. Left bar shows performance on trials with IR light turned on, but no stimulation. The right bar shows the performance from the same sessions for the trials in which we stimulated as usual. Error bars are s.e.m. Data are from 11 sessions in two rats. Figure 2: Rats discriminate among IR sources using graded stimulation frequencies. ( a ) Learning curve for IR-only trials. Graph shows percentage of correct trials as a function of session number (130 sessions in four rats). Black circles/lines indicate mean/s.e.m. for blocks of three sessions. ( b ) Latency decreases as rats learn the task. Scatter plot of latency on IR-only trials, using same conventions as panel a (data are from 66 sessions in two rats). ( c ) Discrimination performance varies with angle between ports. Plot shows percentage of correct trials versus task difficulty (angle between ports). Data are from 100 sessions in two rats. ( d ) Performance degrades when stimulation frequency is constant rather than variable. Plot on the right shows performance on trials in which the stimulation frequency is variable (top left inset) versus held constant (bottom left inset). Data are from 34 sessions in two rats. ( e ) When stimulation is turned off, performance is abolished. Left bar shows performance on trials with IR light turned on, but no stimulation. The right bar shows the performance from the same sessions for the trials in which we stimulated as usual. Error bars are s.e.m. Data are from 11 sessions in two rats. Full size image We performed a series of additional psychophysical tests on the new modality. First, we varied task difficulty by changing the angle between the ports. Moving the ports closer together increased uncertainty about the stimulus source, as the light from each IR source had a broad wavefront ( Fig. 1a ), and the IR detector had a relatively wide ‘receptive field’ (see Methods). While animals consistently performed above 90% of the trials correctly when the ports were 90° apart, this performance dropped off quickly as the angles between the IR sources were reduced below 60° ( Fig. 2c ; Supplementary Movie 3 ). Behavioural performance was significantly dependent upon task difficulty ( P =1.1 × 10 −19 ; analysis of variance). Because the rats swept their heads back and forth to sample the IR signals, we hypothesized that the rats were sensitive to the intensity of IR light, not just its presence or absence. To test this, in some sessions we randomly interspersed trials in which stimulation frequency was held constant, so the animal only received binary information about IR presence ( Fig. 2d , left). Performance was significantly degraded in such constant-frequency trials ( P =0.0001; two-way analysis of variance), demonstrating that the rats were sensitive to graded IR signals ( Fig. 2d , right). Rats are typically considered blind to the IR spectrum [11] : their cone spectral sensitivity is negligible above 650 nm [14] , which is well outside the spectral emission of our IR source (940 nm peak emittance, with a range of non-zero emission between 825 and 1000, nm; see Methods). However, in the sensory prosthetics literature there has been some concern about the true range of spectral visual sensitivity of the rat [15] , so we also experimentally checked whether our animals succeeded by using their visual system to discriminate the IR cues. In two animals we added random ‘no stimulation’ trials in which the IR light turned on, but there was no stimulation delivered to the cortex. Performance on the task was abolished in all 11 sessions, dropping from 69±3.2 to 8±5.2% correct, a significant change ( P =7.6 × 10 −6 ; paired t -test) ( Fig. 2e ). Percent correct was below 33% on the trials without stimulation because in the majority of trials the animals did not poke in any of the ports, and simply let the trial time out (see Online Supplementary Movie 4 ). Analysis of activity in S1 Next, we investigated the effects, within S1, of acquiring the new sensory modality. For instance, are some neurons ‘hijacked’ by IR inputs [16] , such that they no longer respond to whisker stimulation? To address this question, we recorded from multi-electrode arrays chronically implanted in S1 infragranular cortex in two well-trained rats ( N =76 single units over five sessions). We presented three different stimuli, each lasting 200 ms: unilateral whisker deflection (via air puffs), ICMS (using current magnitudes that were applied during the task) and both stimuli delivered simultaneously. S1 neurons were clearly not hijacked by ICMS, even after many months of microstimulation. In fact, most (83%) S1 neurons showed quite robust responses to whisker deflection ( Fig. 3a ). The breakdown of all response types is detailed in Fig. 3c . Briefly, of 76 units, 84% (64/76) responded to one or the other stimulus, while 16% (12/76) showed no significant response to either stimulus. The majority (83% (63/76)) showed significant responses to whisker deflection. Of these, 83% (52/63) were multimodal neurons, exhibiting significant responses to ICMS as well. Only one neuron in our sample showed a response to ICMS but not whisker deflection. Among the multimodal S1 neurons, the response to both stimuli delivered simultaneously was highly sublinear ( Fig. 3d ; P =4.6 × 10 −17 ; two-tailed paired t -test). 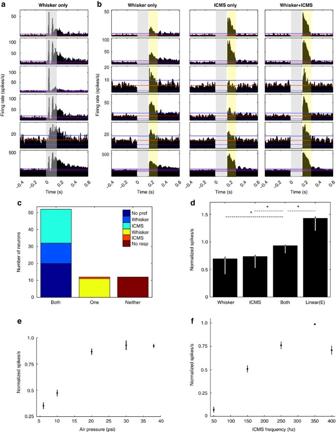Figure 3: Neurons in S1 respond to both whisker deflection and ICMS. (a) Sample peristimulus time histograms from neurons (rows) recorded simultaneously in an anesthetized animal during whisker deflections. The grey strip indicates time of whisker deflection (0–200 ms). Blue/red lines indicate mean± three s.d. values from the mean firing rate during the baseline period before stimulation. Rows 1–5 are single-unit responses, while row 6 is a representative multiunit response. (b) Sample peristimulus time histograms from the same neurons in panelaunder three stimulus conditions. Left column: response to whisker deflection (38 psi air puff), but with the response during stimulation clipped out to enable comparison with the other two columns. Middle column: response to ICMS only (250 Hz). Right panel: response to simultaneous whisker deflection and ICMS. The light yellow strip indicates the time, after stimulation, we used to compare response magnitudes in the three cases. Note there are no responses during electrical stimulation because of electrical artifacts, so the firing rates drop to zero during those epochs. (c) Overall distribution of response types. Columns are segregated by whether neurons responded significantly to both stimuli, only one stimulus, or neither. (d) Mean (+s.e.m./−standard deviation) response of multimodal neurons to each of the three stimuli. The observed response to both stimuli is significantly sublinear (fourth bar indicates expected response under assumption of linearity). Asterisks indicate significance withP<1.0 × 10−6(paired, two-tailedt-test). (e) Multiunit response magnitude (mean firing rate±s.e.m.) as a function of whisker deflection magnitude (intensity of air pressure applied to whiskers) for 16 channels in two animals. Zero is baseline (mean rate before stimulus onset), and responses for each channel were normalized to the maximum mean response over all three stimulus conditions. (f) Multiunit response magnitude versus ICMS frequency, with the same conventions as in panele, with 13 channels in two animals. Figure 3: Neurons in S1 respond to both whisker deflection and ICMS. ( a ) Sample peristimulus time histograms from neurons (rows) recorded simultaneously in an anesthetized animal during whisker deflections. The grey strip indicates time of whisker deflection (0–200 ms). Blue/red lines indicate mean± three s.d. values from the mean firing rate during the baseline period before stimulation. Rows 1–5 are single-unit responses, while row 6 is a representative multiunit response. ( b ) Sample peristimulus time histograms from the same neurons in panel a under three stimulus conditions. Left column: response to whisker deflection (38 psi air puff), but with the response during stimulation clipped out to enable comparison with the other two columns. Middle column: response to ICMS only (250 Hz). Right panel: response to simultaneous whisker deflection and ICMS. The light yellow strip indicates the time, after stimulation, we used to compare response magnitudes in the three cases. Note there are no responses during electrical stimulation because of electrical artifacts, so the firing rates drop to zero during those epochs. ( c ) Overall distribution of response types. Columns are segregated by whether neurons responded significantly to both stimuli, only one stimulus, or neither. ( d ) Mean (+s.e.m./−standard deviation) response of multimodal neurons to each of the three stimuli. The observed response to both stimuli is significantly sublinear (fourth bar indicates expected response under assumption of linearity). Asterisks indicate significance with P <1.0 × 10 −6 (paired, two-tailed t -test). ( e ) Multiunit response magnitude (mean firing rate±s.e.m.) as a function of whisker deflection magnitude (intensity of air pressure applied to whiskers) for 16 channels in two animals. Zero is baseline (mean rate before stimulus onset), and responses for each channel were normalized to the maximum mean response over all three stimulus conditions. ( f ) Multiunit response magnitude versus ICMS frequency, with the same conventions as in panel e , with 13 channels in two animals. Full size image Population responses in S1 increased according to a saturating function of whisker deflection magnitude ( Fig. 3e ). Response magnitudes also increased with ICMS frequency up to 350 Hz, but dropped off at 400 Hz, likely due to adaptation ( Fig. 3f ). This neuronal response-profile is akin to an IR receptive-field for the range of IR stimulation frequencies employed in the task. In 1969, Bach-y-Rita performed the classic ‘sensory substitution’ experiments, in which visual stimuli were projected onto the skin via mechanical actuators, allowing congenitally blind patients to experience a visual world for the first time [4] . Here we have applied the logic of sensory substitution directly to the somatosensory cortex, bypassing the body’s periphery, with the goal of building a cortical sensory prosthesis capable of augmenting the subject’s perceptual capability [5] . Instead of giving a binary, top–down signal instructing the rats where to move [17] , we connected S1 to a new graded sensory cue available in their environment, and they spontaneously adopted novel foraging behaviours in response. Note that, in principle, this experimental paradigm could use any novel stimulus (for example, magnetic or radio waves) to be represented in S1. We observed that neurons in the stimulated regions of S1 maintained their ability to respond to whisker deflection. This suggests that two different cortical representations (one tactile and one IR) became superimposed on the animal’s S1 cortex, creating a novel bimodal processing region. However, it is important to emphasize that behavioural studies will be needed to determine the consequences, for whisker-based tactile discrimination, of adding this new information to S1. The mechanisms by which animals learn to use this new information source will also be an interesting avenue for future research, as such research should suggest how to accelerate sensory prosthetic acquisition. To investigate the mechanisms of plasticity, including those theories implicating glial cells [18] , it will be helpful to examine functional and structural changes in cortical and subcortical tactile processing centres as rats learn to discriminate among IR sources. Overall, our behavioural results suggest that animals initially treated S1 electrical stimulation as an unexpected whisker deflection, and eventually treated it as a stimulus originating away from the body in the surrounding environment. However, we are unable, using the methods in this paper, to determine whether the fully trained rats consciously experienced microstimulation as a new distal sensory modality, or simply learned to associate a tactile sensation with an otherwise imperceptible distal sensory cue. This is a question that could presently be addressed with sensory substitution experiments in humans. Indeed, one such study suggests that some subjects experienced tactile stimuli as visual in nature after training with a visual-to-tactile peripheral substitution device [19] . The next generation of sensory neuroprosthetics research in humans will likely continue to rely on ICMS rather than optogenetics [20] , [21] . Indeed, our experimental strategy has been quite different from optogenetic approaches [22] , [23] , [24] , [25] : instead of stimulating a specific cell-type population, we indiscriminately stimulated all S1 neurons in the vicinity of the stimulating electrodes’ tips. Despite the fact that this unusual signal was delivered at extremely high frequencies, and likely spread through most of S1 [26] , [27] , [28] , these animals readily learned to exploit this new sensory channel. One potential application of the technology used in this study is in the design of a new generation of motor neuroprostheses that, instead of simply sending a brain-derived motor control signal to move a prosthetic limb, would provide continuous sensory feedback to the user’s brain from the prosthesis [29] , [30] , [31] . Such closed-loop bidirectional brain–machine–brain interaction could significantly improve reaction time, behavioural accuracy and likely aid the integration of the limb into the user’s internal body image [9] , [30] , [32] , [33] . However, there is another aspect of the present work that has rarely been explored in the neuroprosthetics literature: the potential to expand or augment a species’ normal perceptual range. In that pursuit, we have implemented, as far as we can tell, the first cortical neuroprosthesis capable of expanding a species’ perceptual repertoire to include the near IR electromagnetic spectrum, which is well outside the rat photoreceptors’ spectral sensitivity. Thus, by taking advantage of this novel paradigm, our rats were able to transcend the limitation of perceiving only those stimuli that can activate their bodies’ native sensory transducers. Behavioural task and training All experiments were performed on female Long Evans rats ~14-weeks-old (~250 g; Harlan Laboratories). Rats were trained in a chamber with three reward ports that were situated 90° apart ( Fig. 1a ). Each port was fit with a visible broad-spectrum LED, and an infrared LED (Opto Semiconductors Inc., 940 nm peak emittance (range of non-zero emissions was between 825 and 1000, nm), and IR intensity dropped to half-max at 120°) ( Fig. 1a ). We first trained water-deprived rats to poke in the port whose visible LED was activated. Each trial began when a visible light in one randomly selected port was activated. Rats received water when they broke the photobeam in that port (correct trials). Trials counted as incorrect when the rats poked in a different port, or did not poke at all and let the trial terminate (this was set to occur between 15 and 20 seconds after the onset of the light). On incorrect trials, they received no water, an error tone, and a longer delay to the next trial. For some rats, we delivered air puffs to the face on incorrect trials. Once animals performed above a criterion value (>70% correct) >4 days in a row, we implanted an array of stimulating electrodes into S1 ( Fig. 1d ). The array includes an IR detector attached to the connector (see Fig. 1c and Surgery below). After the animals recovered from surgery, we determined the minimal currents required to evoke a behavioural response in at least two electrode pairs (thresholds were between 1 and 200 μA, see Stimulating Electrodes and Stimulator below for details). We then trained them in the same behavioural chamber, but incrementally replacing visible light with ICMS linked to IR levels from their detector ( Fig. 1e ). Initially, each trial had the same structure as trials in the initial behavioral task described above, except that the onset of the visible light was preceded by IR-level dependent stimulation (up to 400 Hz) that lasted 0.6–1.5 s. In four of six rats, we began with brief durations of stimulation (600–700 ms) to acclimate them to stimulation. In two of the rats, we started with longer stimulation durations to get estimates of behavioural latency as they learned the task ( Fig. 2b ). Thus the animals learned that stimulation indicated the presence of the visible light. The stimulation frequency was exponentially proportional to the IR levels ( Fig. 1e ). We used an exponential function because IR intensity dropped logarithmically from the IR source. We stimulated at high frequencies for two reasons: one, in preliminary experiments we found that using a lower frequency range (that is, 0–100 Hz) yielded less reliable performance; two, we wished to avoid evoking kindling seizures [34] . Stimulation frequencies were updated every 50 ms based on IR levels, and it took ~5 ms for the stimulation frequency to actually change in the rat once the command was sent. Pulse frequency was the only variable that tracked IR levels: current amplitudes were kept the same for each pulse. Once it became clear, based on visual inspection, that the animals were comfortable with stimulation, we added ‘IR-only’ trials in which the IR-dependent stimulation would appear without any accompanying visible light. That is, on these IR-only trials they could only use the signals from ICMS to get to the correct port. They trained on this until their performance on the IR-only trials reached a criterion value of 70% correct. For some rats that stayed above criterion for four sessions in a row, we then varied task difficulty in which across sessions, we pseudo-randomly chose a new angle between the ports (either 90, 60, 45 or 30 degrees; Fig. 2c ). On some sessions, we added a small percentage of trials (~15%) in which the stimulation frequency was held constant, regardless of the IR intensity. Such constant-frequency trials allowed us to compare performance when the stimulation frequency depended on IR levels with those trials when stimulation frequency was a constant function of IR intensity ( Fig. 2d , left hand side). All behaviour control was run in custom Matlab scripts using the data acquisition toolbox (run with NIDAQ PCI-7742 card, National Instruments). Stimulating electrodes and stimulator In preliminary studies, we found that the thresholds for evoking behavioural responses were lower with electrode pairs within the same penetration of the cortex. Hence, for each biphasic stimulating electrode, we joined pairs of 30-μm stainless steel microwires to one another, each pair separated by 300 μm ( Fig. 1c inset). We attached a single infrared detector (Lite-On Inc) to the connector (Omnetics), and powered the IR detector through the two extra reference pins on the connector. The phototransistor in the detector had a peak spectral sensitivity at a wavelength of 940 nm. The range of sensitivity was from 860 to 1020, nm, and its ‘receptive field’ (that is, the angular range within which a 940 nm test stimuli would evoke a response from the detector) was 20° in diameter at half-max ( Fig. 1a ). We used bipolar stimulation with charge-balanced, biphasic pulse trains, using a custom-controlled stimulator, as described elsewhere [35] . Pulses were 100 μs in duration, with 50 μs between the cathodic and anodic phases of the pulses ( Fig. 1e ). Current magnitudes varied between 1 and 300 μA. Before training rats on the IR-version of the task, we determined current thresholds by placing them in the empty behavioural chamber ( Fig. 1a ), and stimulating with 1 μA at 200 Hz for 500 ms. If an animal noticeably moved in response to stimulation (this typically involved locomoting, moving their heads to the side or scratching at their faces), that current level was taken as the threshold current. If not, we increased the current amplitude by 50%, keeping the frequency and duration the same, until we noted such a response. We used electrical microstimulation in lieu of optogenetics in this study, as one goal is to integrate this technology into human studies in the near future (see Discussion). Surgery Detailed surgical procedures are described elsewhere [36] . Briefly, we implanted the stimulating electrodes into S1 (−2.5 mm posterior and 5.5 mm relative to bregma, 1.5 mm deep) under pentobarbital anaesthesia (0.065 mg g −1 ), and the rats were given at least a week to recover from the surgery before being deprived again. The Duke University Institutional Animal Use Committee approved all surgical and behavioural methods. Neural recording and sorting The basic recording set-up is described in detail elsewhere [36] . Namely, on those channels that we were not using for stimulation, we recorded neural activity using the (Multichannel Acquisition Processor (Plexon, Inc., Dallas, Texas)). To stimulate and record simultaneously without damaging the head stage, we peeled off the wires connected to the stimulator from the connector to bypass the head stage, while the other channels went directly to the head stage. Sorting of neural data is also described elsewhere [36] . Briefly, in addition to template-based online sorting, all voltage traces around a threshold-crossing event were saved for offline sorting. For offline sorting, we used clustering in principal component space, signal to noise ratio and autocorrelation functions that showed a clear absolute and relative refractory period to determine whether the data came from single units or multiple units. In our recordings, we lightly anesthetized head-fixed animals under isofluorane anaesthesia (0.8–3% isofluorane mixed with pure oxygen). We controlled the duration and magnitude (psi) of air via a modified fluid dispenser (Oki DX-250, Garden Grove, CA), which was controlled with TTL pulses sent from Matlab. Before recording, we positioned the air dispenser to stimulate the majority of the large whiskers, ~10 mm from the whisker pad. We delivered three different stimuli, in pseudo-random order: air puff to whiskers, electrical stimulation and both stimuli delivered simultaneously (see Fig. 3 ). Statistical methods We calculated significant responses in peristimulus time histograms using a bootstrap cumulative sum algorithm described in more detail elsewhere [37] . This involved taking bootstrap samples of the cumulative response during a baseline period (period before time zero in Fig. 3a ), and using these to generate a cumulative sum 95% confidence interval (with Bonferonni correction for multiple comparisons), and comparing this to the actual cumulative sum during the period of stimulation. A significant response was when the actual cumulative sum left the 95% confidence interval, and ended when the response dropped below a 95% confidence interval estimated from bootstrapping the original data. During electrical stimulation, recordings were saturated by stimulus artifact, so to directly compare responses between whisker deflection and ICMS, we compared mean firing rates during the 130 ms period following the offset of both stimuli. To compare relative response magnitudes among multiple neurons, we normalized the mean response to each stimulus by the maximum mean response over all three stimulus conditions, so the maximum response was assigned a value of one. To generate the predicted responses to both stimuli delivered simultaneously ( Fig. 3c ), we used the normalized responses described in the previous paragraph. For a linear system, the predicted response to both stimuli would simply be the sum of the responses to each stimulus taken individually. That is, R ( E + W )= R ( E )+ R ( W ), where E is electrical stimulation, W is whisker deflection, and R ( x ) signifies the response to input x . How to cite this article: Thomson, E.E. et al . Perceiving Invisible Light through a Somatosensory Cortical Prosthesis. Nat. Commun. 4:1482 doi: 10.1038/ncomms2497 (2013).